The reverse evolution from multicellularity to unicellularity during carcinogenesis Theoretical reasoning suggests that cancer may result from a knockdown of the genetic constraints that evolved for the maintenance of metazoan multicellularity. By characterizing the whole-life history of a xenograft tumour, here we show that metastasis is driven by positive selection for general loss-of-function mutations on multicellularity-related genes. Expression analyses reveal mainly downregulation of multicellularity-related genes and an evolving expression profile towards that of embryonic stem cells, the cell type resembling unicellular life in its capacity of unlimited clonal proliferation. Also, the emergence of metazoan multicellularity ~600 Myr ago is accompanied by an elevated birth rate of cancer genes, and there are more loss-of-function tumour suppressors than activated oncogenes in a typical tumour. These data collectively suggest that cancer represents a loss-of-function-driven reverse evolution back to the unicellular ‘ground state’. This cancer evolution model may account for inter-/intratumoural genetic heterogeneity, could explain distant-organ metastases and hold implications for cancer therapy. Unicellular life appeared first on the Earth, followed by multicellular life as a result of selection for cooperation between the unicellular individuals [1] . Complex multicellular organisms, including humans, possess sophisticated regulatory pathways that may be viewed as genetic mechanisms suppressing the fitness of individual cells to ensure the fitness of the whole organism [2] , [3] . However, events such as somatic mutations or viral infections may eradicate such constraints and reactivate a cell’s otherwise dormant capacity of seeking its own fitness, resulting in cancer [4] , [5] , [6] . In this regard, cancer can be viewed as a reversal of the macroevolution from unicellular life to multicellular life [7] , [8] , [9] . This reasonable conjecture has important implications for cancer research, prevention and therapy, but has never been tested rigorously. To address this question, we carried out experimental evolution [10] , [11] of a human breast cell-derived xenograft tumour in mice to characterize the complete evolutionary history of a tumour. Although the micro-environment of the mouse mammary gland is not ideal for studying human breast cancer, such a strategy has long been used in the cancer community [12] , and has been proven to be highly successful in human cancer biology [13] . We observed a generally loss-of-function strategy to knockdown the genetic constraints required for the maintenance of multicellularity during cancer evolution. An experimental evolution of a xenograft tumour Similar to the pioneer study [14] , we engineered a mutated version of the human oncogene HRAS V12 into the otherwise normal immortalized human breast epithelial cell line MCF10A, to obtain an early transformed cell population MCF10A- HRAS . MCF10A- HRAS cells were subsequently xenografted into NOD/SCID mice to form the first-stage xenograft tumour (XT1). The cell population of the XT1 was then xenografted again to build the second-stage xenograft tumour (XT2). This procedure was repeated until two metastatic tumours were observed in the mouse carrying XT8 ( Supplementary Fig. 1 ). Cell samples from MCF10A- HRAS , XT1, XT2, XT3, XT4, XT5, XT6, XT7, XT8, and the two metastatic tumours XT8_M1 and XT8_M2 are in clear temporal order, collectively representing the tumour’s full-life history from initiation to metastasis. We then performed comparative genomic hybridization ( Supplementary Data 1 ), high-depth (~250X) exome sequencing ( Supplementary Data 2 ) and RNA sequencing ( Supplementary Data 3 and Supplementary Fig. 2 ) on each of the cell samples and built the first high-time-resolution evolutionary roadmap of a tumour at the genomic and transcriptomic levels. The temporal distribution of intratumoural heterogeneity We detected 473 single-base substitution mutations that originated after XT1, with each showing varied allele frequencies at different tumour stages ( Supplementary Data 2 ). We grouped mutations whose frequencies varied in a similar manner and identified five major mutation groups that together represent diverse subclones, which we validated by single-cell analysis ( Supplementary Data 2 ). One subclone constituted a minor fraction of cells while harbouring the vast majority of detected mutations after XT4 ( Fig. 1a ), suggesting that it is a mutator. In this subclone, we observed missense mutations on MLL3 and RAD54B , two genes required for maintaining genome stability, at XT4 and subsequent stages, as well as a missense mutation on PMS1 , a gene involved in DNA mismatch repair, starting at XT7 ( Fig. 1b ), consistent with the identification of this subclone as a mutator and explaining the pattern of increased mutations in this subclone ( Fig. 1a ). Interestingly, the two metastases, XT8_M1 and XT8_M2, were both seeded by this mutator subclone ( Fig. 1a and Supplementary Fig. 3 ), an observation reminiscent of the long-standing hypothesis that mutator phenotypes promote cancer evolution [15] . 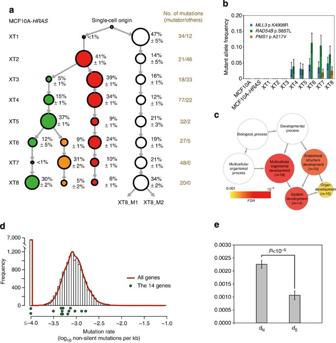Figure 1: The evolving intratumoural genetic heterogeneity reveals positive selection on a set of multicellularity-related genes. (a) The expansion or contraction of intratumoural subclones during the experimental evolution. The area of a circle is proportional to the cell frequency of the subclone, which is two times the average allele frequency of mutations found in the subclone and shown next to the circle (mean±s.e.m.). The unfilled circle represents the subclone that became a mutator after XT4. The numbers of mutations observed in the mutator subclone and in remaining parts of the tumour are shown at the left. (b) Allele frequencies of the three missense mutations onMLL3,RAD54BandPMS1. (c) GO terms enriched with genes mutated in the mutator subclone. Arrows stand for ‘is_a’, and FDR is false discovery rate. The number of mutated genes in each GO term is shown inside each circle. (d) The rates of non-silent mutations (missense, nonsense, and splicing-altering substitutions as well as indels) for each of the 14 multicellularity-related genes with non-synonymous mutations in the mutator subclone and for all human protein-coding genes in a total of 772 breast cancer samples in TCGA. (e)dN>dS, a signature of positive selection on the 14 genes in breast cancer clinical samples. The error bar shows one s.e. Figure 1: The evolving intratumoural genetic heterogeneity reveals positive selection on a set of multicellularity-related genes. ( a ) The expansion or contraction of intratumoural subclones during the experimental evolution. The area of a circle is proportional to the cell frequency of the subclone, which is two times the average allele frequency of mutations found in the subclone and shown next to the circle (mean±s.e.m.). The unfilled circle represents the subclone that became a mutator after XT4. The numbers of mutations observed in the mutator subclone and in remaining parts of the tumour are shown at the left. ( b ) Allele frequencies of the three missense mutations on MLL3 , RAD54B and PMS1 . ( c ) GO terms enriched with genes mutated in the mutator subclone. Arrows stand for ‘is_a’, and FDR is false discovery rate. The number of mutated genes in each GO term is shown inside each circle. ( d ) The rates of non-silent mutations (missense, nonsense, and splicing-altering substitutions as well as indels) for each of the 14 multicellularity-related genes with non-synonymous mutations in the mutator subclone and for all human protein-coding genes in a total of 772 breast cancer samples in TCGA. ( e ) d N > d S , a signature of positive selection on the 14 genes in breast cancer clinical samples. The error bar shows one s.e. Full size image Positive selection on a few multicellularity-related genes To understand what properties enabled the mutator subclone to seed the metastases, we studied the 137 genes that are mutated in the mutator subclone (from XT4 to XT8) using Gene Ontology (GO) analysis. We found that they are enriched exclusively in four closely related GO terms under a false discovery rate of 0.001 ( Fig. 1c ). The enrichment signal remained largely the same for a subset of genes with substantial expression in the cell populations ( Supplementary Fig. 4 ). We observed no significant GO enrichment for genes mutated in other subclones. Among the four GO terms, ‘systems development’ and ‘organ development’ are children of the two highly similar sibling terms ‘multicellular organismal development’ and ‘anatomical structure development’, which share ~90% of genes with each other. Because anatomical structure is apparently a feature specific to multicellular organisms, all of these GO terms were thus considered to be multicellularity-related. We examined the 15 mutated genes shared between the two sibling terms ‘multicellular organismal development’ and ‘anatomical structure development’ and found 14 non-synonymous (missense and nonsense) mutations and 1 synonymous mutation, whereas we observed 81 non-synonymous mutations and 43 synonymous mutations on the other 122 genes mutated in the mutator subclone, suggesting that the 15 multicellularity-related genes tend to show functional changes ( P <0.04, two-tailed Fisher exact test). We ignored the single gene carrying no non-silent mutation, leaving the 14 other genes for further examination ( Supplementary Table 1 ). None of the 14 genes belong to the ~500 cancer drivers annotated by the Cancer Gene Census (CGC) [16] , and, in line with this, they are mutated only at background frequency in breast cancer clinical samples ( Fig. 1d ). Interestingly, however, from a total of ~800 sequenced exomes of breast cancer clinical samples we observed 220 non-synonymous mutations and 37 synonymous mutations on the 14 genes, corresponding to an overall d N / d S =2.13 ( P <10 −5 , Binomial test; Fig. 1e and Supplementary Data 4 ), where d N stands for the number of non-synonymous mutations per non-synonymous site, and d S stands for the number of synonymous mutations per synonymous site. This result is not due to a single outlier gene, because the d N / d S ratio remained largely unchanged (varying from 1.85 to 2.22) after removing any one of the 14 genes, suggesting that the 14 multicellularity-related genes are overall under positive selection in breast cancer. We noted that their tendency towards function-altering mutations appears to be stronger in our xenograft model (14:0) than in the clinical samples (220:37), although the difference is not statistically significant ( P =0.23, two-tailed Fisher exact test). We speculated that the functional alterations of the 14 genes may directly contribute to metastasis, such that the signal from the metastasis-seeding subclone in our xenograft model is stronger than the signal from the clinical samples, which were mostly whole primary tumours containing non-metastasizing cancer cells that dilute the signal. We examined ~100 genome-wide screens for mutations in metastatic tumours and discovered 82 non-synonymous mutations and 6 synonymous mutations on the 14 genes ( Supplementary Data 4 ). Thus, comparison of the two groups of clinical samples suggests that the tendency to have function-altering mutations is indeed stronger in metastatic tumours ( P =0.04, one-tailed Fisher exact test), a result well in line with our hypothesis that positive selection on the 14 genes drives metastasis. Notably, in addition to 16 nonsense mutations, the 300 missense mutations examined here are distributed along the entire length of each of the 14 genes without apparent hotspots ( Supplementary Fig. 5 ), suggesting that, in general loss of function is positively selected [17] , although rare gain-of-function mutations may exist. An evolving expression profile towards unicellularity We identified 12,911 genes that show marked expression changes during tumour evolution. Analogous to the concept of driver mutations and passenger mutations, these changes should include both driver expression changes (DEC) and passenger expression changes (PEC). We reasoned that, compared with DECs that are beneficial to tumour cells, PECs subject to further expression reprogramming are less likely to have fitness costs, such that the PEC genes tend to show both increasing and decreasing expression during the tumour’s life history. With this logic in mind, we developed an algorithm and detected the PEC signature for the vast majority (~95%) of genes with marked expression changes. The remaining ~700 genes show largely one-way changes (that is, either exclusively increasing or exclusively decreasing), and thus are likely to have undergone DECs ( Supplementary Data 3 ). 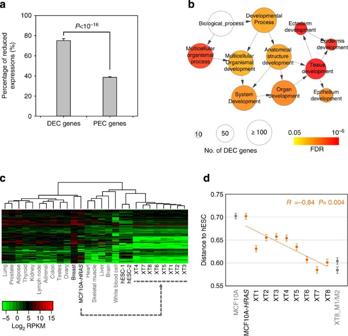Figure 2: Properties of the gene expression evolution during carcinogenesis. (a) The percentage of reduced expression levels for putative DEC (driver expression change) and PEC (passenger expression change) genes, respectively. The error bar shows one s.e. (b) The putative DEC genes are enriched in multicellularity-related GO terms. Arrows stand for ‘is_a’, and FDR is false discovery rate. (c) Expression evolution of the 73 DEC genes preferentially expressed in the breast. (d) An evolving expression profile approaching that of ES cells was observed when all of the 12,911 genes with marked expression changes were examined. The distance (y-axis) was measured by 1-Rho^2, whereRhois the Spearman correlation coefficient of two expression profiles. Consistently, gene set enrichment analysis (GSEA) [18] showed that the ~700 genes with putative DECs are involved in a large number of known cancer-related pathways/processes ( Supplementary Table 2 ). We found that up to 75.1% of these genes show reduced expression levels, while only 38.6% of genes with the PEC signature are downregulated ( P <10 −16 , χ 2 -test; Fig. 2a ), suggesting a ‘less is more’ pattern in cancer driver expression divergences. A particularly interesting observation is that, similar to the genes that are mutated in the mutator subclone ( Fig. 1c ), the putative DEC genes are also overrepresented in a series of multicellularity-related GO terms ( Fig. 2b ). Although inactivation of a specific gene can either strengthen or weaken a cellular process, the widespread shutting down of the genes necessary for development and maintenance of multicellularity suggests a general loss-of-function strategy to erase the cellular features of multicellularity during cancer. Figure 2: Properties of the gene expression evolution during carcinogenesis. ( a ) The percentage of reduced expression levels for putative DEC (driver expression change) and PEC (passenger expression change) genes, respectively. The error bar shows one s.e. ( b ) The putative DEC genes are enriched in multicellularity-related GO terms. Arrows stand for ‘is_a’, and FDR is false discovery rate. ( c ) Expression evolution of the 73 DEC genes preferentially expressed in the breast. ( d ) An evolving expression profile approaching that of ES cells was observed when all of the 12,911 genes with marked expression changes were examined. The distance ( y -axis) was measured by 1- Rho^2 , where Rho is the Spearman correlation coefficient of two expression profiles. Full size image Some of the ~700 putative DEC genes are ubiquitously expressed in diverse normal tissues, while some are preferentially expressed in the breast. We next looked specifically at the evolution of the putative DEC genes preferentially expressed in the breast. Following a previous study [19] , we calculated a breast biased index (BBI) for each of the ~700 putative DEC genes by dividing its expression level in the breast by its median expression level in all 16 normal tissues, obtaining 73 genes with BBI>2 ( Supplementary Data 5 ). We clustered the expression profiles of these 73 genes based on the pairwise Euclidean distance of these tissues or cells. MCF10A- HRAS , the starting cell population, clustered with the normal breast tissue; interestingly, the latter XT cell populations are all clustered with embryonic stem (ES) cells ( Fig. 2c ). We were unable to capture any intermediate statuses because the distance calculation based on the 73 genes has large variations that prevent comparisons among the XT cell populations ( Supplementary Fig. 6 ). However, we successfully observed a gradually evolving trend towards ES cells when the profile of all differentially expressed genes was used ( Fig. 2d ). In addition to their totipotency, an often underappreciated characteristic of ES cells is their excessive proliferation to produce functionally equivalent progeny, a feature typical to unicellular life. It seems more reasonable that the unicellularity, rather than the totipotency, of ES cells is mimicked by the XT cell populations during tumour evolution. Elevated birth rate of cancer genes on deep metazoan branches Our findings from the experimental evolution of a breast tumour appear to be consistent with the hypothesis that cancer evolves via knockdown of the genetic network of multicellularity. It was next important to determine whether this idea applies to clinical data from various cancers. We reasoned that the formation of the genetic network required for the development and maintenance of multicellularity in humans following the origin of metazoan multicellularity involved the co-option of some pre-existing genes and the gradual acquisition of other new genes during the course of evolution. It is conceivable that genes originating at the emergence of metazoan multicellularity should have a higher probability of contributing to the core multicellularity-related genetic network. If cancer is indeed driven by demolishing this network, one would expect that genes born at the emergence of metazoan multicellularity will present an elevated likelihood of being cancer drivers. This prediction is favoured by a previous phylostratigraphy analysis that showed an elevated birth rate of cancer-related human genes on the branch connecting Holozoa and Metazoa [20] . The result, however, might have been confounded by the then-confusing phylogeny of deep animal clades and the underrepresentation of fast-evolving genes in deep branches. As cancer drivers are evolutionarily more conserved than other human genes ( Supplementary Fig. 7 ), it is important to control for gene conservation in the analysis. We assembled 37 completely sequenced genomes representing 13 major clades ( Fig. 3a and Supplementary Data 6 ), conducted all-against-all protein BLAST for 37*36/2=666 species pairs, and built an orthology network in OrthoMCL [21] that solves gene orthologous relationship using graph theory. We successfully dated the origin of ~21,000 human genes, including 488 cancer drivers annotated by the CGC. As a control, we performed a simulation by randomly picking 488 genes with evolutionary rates comparable to the 488 cancer drivers to derive the null distribution. We ran the simulation 13,000 times and found that genes originating on the Branch #3 (or B3) include significantly more cancer drives than expected ( P <0.01 after Bonferroni correction; Fig. 3b ). Branch #2 (B2) is a long branch connecting unicellular life with the oldest multicellular lineage, Ctenophora ( Fig. 3a ), and shows a slightly weaker signal ( P =0.05 after Bonferroni correction; Fig. 3b ). We reason that this signal might have been diluted, as genes first observed in Ctenophora could have been born far earlier than the emergence of metazoan. Inclusion of more genomes on B2 would help to resolve this issue [20] . At any rate, the observation of an increased proportion of cancer drivers on the two deepest metazoan branches clearly supports the argument that cancer can be considered as a process of destroying the genetic network that evolved for the development and maintenance of multicellularity. 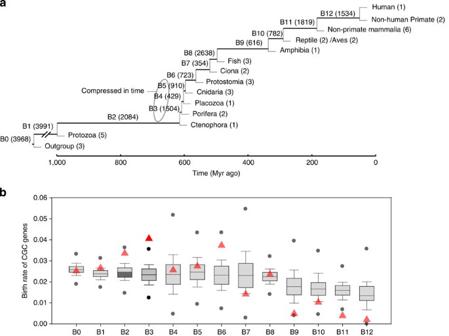Figure 3: The birth rate of cancer drivers peaked on the deepest branches of metazoans. (a) The phylogenetic relationships of humans and the 13 major clades. Emergence of the four early metazoan clades, Ctenophora, Porifera, Placozoa and Cnidaria, was extremely compressed in time ~600 Myr ago. The number of born genes is shown in parentheses behind each branch, and the number of genomes used for analysis is shown behind each clade. (b) The birth rate of cancer drivers and pseudo-cancer drivers (y-axis), randomly selected genes with evolutionary rates comparable to cancer drivers, on each of the 13 branches (x-axis). Red triangles represent cancer drivers, and box plots represent pseudo-cancer drivers, with horizontal lines showing the median rates and black dots showing the 10th or the 12,990th rates of a branch out of 13,000 simulations. Figure 3: The birth rate of cancer drivers peaked on the deepest branches of metazoans. ( a ) The phylogenetic relationships of humans and the 13 major clades. Emergence of the four early metazoan clades, Ctenophora, Porifera, Placozoa and Cnidaria, was extremely compressed in time ~600 Myr ago. The number of born genes is shown in parentheses behind each branch, and the number of genomes used for analysis is shown behind each clade. ( b ) The birth rate of cancer drivers and pseudo-cancer drivers ( y -axis), randomly selected genes with evolutionary rates comparable to cancer drivers, on each of the 13 branches ( x -axis). Red triangles represent cancer drivers, and box plots represent pseudo-cancer drivers, with horizontal lines showing the median rates and black dots showing the 10th or the 12,990th rates of a branch out of 13,000 simulations. Full size image Loss-of-function-dominant evolution in tumours of patients There are two groups of cancer drivers, oncogenes and tumour suppressors. The former drives cancer mostly by gain-of-function, and the latter by loss-of-function. There are currently a comparable number of oncogenes and tumour suppressors characterized by the CGC. Interestingly, investigation of thousands of clinical samples showed that the number of inactivated tumour suppressors often exceeds that of activated oncogenes when a single tumour is considered (the former is ~2.3 fold-higher than the latter in a typical solid tumour) [17] . This number should still be an underestimation because a large number of genes normally required for the maintenance of multicellularity are expected to be unrecognized minor tumour suppressors. Motivated by this prediction, we developed a new statistical test, namely, d T / d S ratio test, to compute the relative truncating substitution mutation rate ( d T ) to the synonymous substitution mutation rate ( d S ) in cancer. Observation of d T / d S ratios significantly higher than one indicates positive selection for null mutations, which is a unique signature of tumour suppressor genes. The design of the d T / d S test circumvents the problem of low specificity caused by among-gene mutation heterogeneity, a major flaw of conventional computational methods [22] , while maintaining high sensitivity in principle. Indeed, this test performed better than the classical d N / d S test in recovering 10 well-known tumour suppressors ( Fig. 4a ), but detected, under a false discovery rate of 0.1, no significant signal on ~400 olfactory receptors that seem unrelated to cancer ( Fig. 4b ). Using this new method, we analysed data from The Cancer Genomic Atlas (TCGA) and successfully identified as many as 134 novel putative tumour suppressors under a false discovery rate of 0.1 ( Supplementary Table 3 ), a finding reminiscent of a recent study [23] and challenging the view that the growth of the cancer gene list has reached a plateau [17] . It is conceivable that most of the newly identified tumour suppressors are minor cancer drivers, conferring small fitness advantages in primary tumours. Because of clonal interference [24] in which large-effect beneficial mutations suppress small-effect beneficial mutations in an asexual population, minor cancer genes may become effective primarily at late stages of cancer evolution when the pool of large-effect beneficial mutations becomes shallow, suggesting their roles in promoting malignancy or metastasis. Of particular interest is the fact that the 134 novel tumour suppressors are enriched exclusively in the same four multicellularity-associated GO terms as shown in Fig. 1c ( Fig. 4c ). 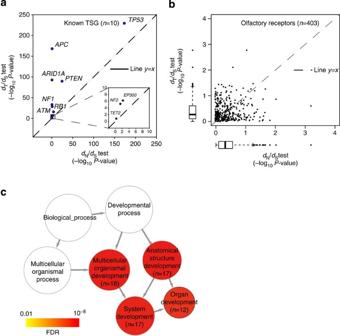Figure 4: Identification of novel tumour suppressors using thedT/dSratio test. Comparison of thedN/dStest and thedT/dStest in detecting positive selection on the ten canonical tumour suppressor genes (a) or on the 403 olfactory receptor genes that seem unrelated to cancer (b). Pooled mutations from 4,506 tumour samples of 13 cancer types were analysed. (c) The 134 novel tumour suppressors are enriched exclusively in the same four multicellularity-related GO terms as inFig. 1c. The number of novel tumour suppressors in each GO term is shown in parentheses. FDR stands for false discovery rate. Figure 4: Identification of novel tumour suppressors using the d T / d S ratio test. Comparison of the d N / d S test and the d T / d S test in detecting positive selection on the ten canonical tumour suppressor genes ( a ) or on the 403 olfactory receptor genes that seem unrelated to cancer ( b ). Pooled mutations from 4,506 tumour samples of 13 cancer types were analysed. ( c ) The 134 novel tumour suppressors are enriched exclusively in the same four multicellularity-related GO terms as in Fig. 1c . The number of novel tumour suppressors in each GO term is shown in parentheses. FDR stands for false discovery rate. Full size image A caveat of this study is that only a single tumour life history was examined, so some of the observed patterns may be rules, while others could be exceptions. Importantly, the two major findings from the experimental evolution are well supported by data from clinical samples or from other studies, suggesting the generality of our results: (1) the metastasis-driving positive selection on the small set of multicellularity-related genes was first suggested by mutations in the experimental evolution and then systematically demonstrated by data from hundreds of clinical samples; and (2) the putative DEC genes were identified based on their one-way expression changes during the experimental evolution and may contain false positives. However, this should have diluted their overrepresentation in known cancer gene sets. In addition, using an isogenically matched cell model with three oncogenes added sequentially so as to mimic the expression divergences during cancer, a previous study found that ~80% of the differentially expressed genes are downregulated [25] . We analysed these genes and found that they are highly enriched in multicellularity-related GO terms ( Supplementary Fig. 8 ), paralleling the findings from the experimental evolution in this study. The idea of cancer as an evolutionary process was first coined by Nowell ~40 years ago [26] . This landmark paper distinguished cancer from genetically inherited diseases that result from a stable mutated genome, providing a basic theoretical framework to guide cancer research and cancer therapy. Notably, cancer cells resemble unicellular life in many of their hallmarks [27] , including sustaining proliferative signalling, evading growth suppressors, resisting cell death and enabling replicative immortality. Although solid tumours are not unicellular entities as far as physical structure is concerned, they are evolving towards a functional status wherein individual cells selfishly seek their private fitness, the essence of unicellular life. Given that the entire cellular machinery necessary for unicellular life is already available in a human cell, cancer may reactivate the otherwise dormant pre-existing functions by knocking down the genetic constraints required for the maintenance of multicellularity. Such a concept is actually quite obvious to evolutionists from a theoretical perspective [7] , [8] , [9] , [28] , but rigorous tests and systematic demonstrations based on experimental/clinical data are lacking. In this article, we assembled various lines of empirical evidence to support the theoretical conjecture that cancer cells evolve back towards unicellularity. There are also several unique features in cancer reverse evolution that are worth discussing. First, although gain of new function is sometimes necessary, for example, to initiate transformation [29] , reverse evolution can be driven by the beneficial loss of function [30] , [31] of existing genes that are numerous in the human genome. Considering that loss-of-function mutations are often much more accessible than gain-of-function mutations [32] , reverse evolution via loss of function seems to be a highly efficient strategy for cancer given its short-term time frame [33] . Indeed, loss-of-function genetic or expression alterations were predominant in the experimental data of this study as well as clinical samples [17] . Thus, the model of reverse evolution driven mainly via loss of function challenges the view that cancer progresses to build a new genetic network; instead, it progressively demolishes the existing multicellularity-related genetic network to reactivate the ‘genetic memory’ of being unicellular [8] . This has important implications for thinking of the evolutionary contingency and convergence in cancer, explaining well the enormous inter-/intra-tumoural genetic heterogeneity observed in the clinic [34] , [35] , [36] , as there can be numerous means of knocking down a system. Second, it is difficult to explain the origin of distant-organ metastasis within a primary tumour by the conventional Darwinian selection model because the metastatic site is often very different from the primary site in cell-biological requirements [37] . We reason that, to establish a distant-organ metastasis, cells of a primary tumour need to shut down genes that respond to signals specifying the cells’ tissue identity, which is exactly the direction of reverse evolution back to unicellularity. Thus, distant-organ metastasis represents a very late stage of reverse evolution, which is internally driven by the loss of multicellularity-associated constraints. Primary tumour formation and metastatic colonization are therefore unified by the same reverse evolutionary process. It is worth pointing out that there seem to be no major genes (like TP53 for primary tumours) that are frequently mutated to promote metastatic colonization in clinical samples [38] , suggesting that the capacity of metastasizing is a complex trait governed by a large number of mutations/genes that are either large-effect with low frequency or small-effect with high frequency. This possibility calls for a quantitative genetic approach to map metastasis drivers [39] . It should be emphasized that we here argue for reverse evolution during cancer as far as the basic features of multi-/unicellularity are concerned. It is, of course, impossible that cancer cells degenerate to become the primitive ancestor living over 600 Myr ago. While the model of reverse evolution via loss of function offers a general theoretical framework for understanding cancer, we are fully aware that it is certainly not the full story of such a complex disease, and many cancer-related processes, such as angiogenesis, immune evasion and tissue infiltration, may rely on evolutionary innovations rather than simple degeneration. Separation of such innovative processes from degenerative processes will be critical for designing effective cancer therapies, as attempts to stop an ongoing degeneration towards the unicellular ‘ground state’ seem unlikely to succeed. Six-week-old NOD/SCID female mice were used in the xenograft experiment, and all experiments involving animals were performed in the Animal Center of SYSU, in accordance to the guidelines of the centre. The 10-stage cell populations A DNA fragment containing HRAS V12 (ref. 40 ), an internal ribosome entry site (IRES), and the coding sequence of green fluorescent protein (GFP) was inserted into the vector pBABE-puro [41] to form pBABE-puro - HRAS V12 , the sequence of which was then verified by Sanger sequencing. This construct was introduced into the immortalized human breast cell line MCF10A, which was purchased from ATCC, using a retrovirus following the standard protocol. GFP-positive cells were selected by flow cytometry, resulting in the MCF10A- HRAS cell population. Approximately 5 × 10 6 MCF10A- HRAS cells were injected into the abdominal mammary fat pad of each of three six-week-old female NOD/SCID mice. One mouse developed a xenograft tumour about 2 months later, which was harvested after 2 months at a diameter of ~2 cm and designated as XT1. The tumour was dissected into small pieces, and suspended in pre-warmed digesting solution, prepared by adding 0.1 mg ml −1 DNase I (Sigma DN25), 0.1 mg ml −1 HAse (Sigma H6254), 5 mg ml −1 Collagenase IV (Sigma C5138) and 10% FBS (Gibco C20270) to DMEM-F12 (Gibco 11330-032). After a 2-h digestion at 37 °C, the product was washed with PBS and then cultured in DMEM-F12 with 50% FBS at 37 °C, in an incubator with 5% CO 2 . About 10 7 to 10 8 adherent cells were harvested 2 days later. We used a 40 μg ml −1 biotin-labelled Anti-Mouse H-2K[d] antibody (BD 553564) to label contaminating mouse cells and subsequently depleted these with Dynabeads Biotin Binder (Life Technology 11047). The resulting XT1 cell population was used for further xenografting, DNA and RNA extraction, and liquid nitrogen stock preparation. The other XT cell populations were obtained through a similar procedure. The immortalized MCF10A and MCF10A- HRAS cells were cultured in DMEM-F12 containing 5% Horse Serum (Gibco 16050-122), and with supplements of 20 ng ml −1 EGF (Gibco PHG0311), 0.5 mg ml −1 hydrocortisone (Sigma H0888), 100 ng ml −1 cholera toxin (Sigma C8052) and 10 μg ml −1 insulin (Sigma I1882). As most of the above supplements were no longer required for the transformed XT cells, all XT cells were cultured in DMEM-F12 containing 10% FBS, with none of the above supplements. This change has minimal effect on gene expressions, as evidenced by the highly similar expression profiles of XT1 cell populations growing in the two media (Pearson’s R =0.98, P <10 −16 ; Supplementary Data 7 ). Comparative genomic hybridization Genomic DNA was extracted from ~5 × 10 6 cells using the DNeasy Kit (Qiagen 69504) and digested by NspI (NEB R0602L) or StyI (NEB R0500L). Adaptors were ligated to the DNA fragments for PCR amplification. The amplified DNA was labelled with biotin using the Affymetrix Genome-Wide Human SNP Nsp/Sty Assay Kit 6.0 (Affymetrix 901015). Hybridization was performed according to Affymetrix Genome-Wide Human SNP Nsp/Sty 6.0 User Guide (Affymetrix 702504). Arrays were then scanned by a GeneChip Scanner 3000 (Affymetrix). The genotype and copy number of each probe or genomic segment were calculated by Genotyping Console Software 4.1 (Affymetrix). These data are presented in Supplementary Data 1 . Exome sequencing Genomic DNA was extracted from ~5 × 10 6 cells using the DNeasy Kit (Qiagen 69504) and sheared by Covaris. Fragments between 200 and 300 bp were collected for library construction following the TruSeq DNA Guide (Illumina). The genomic DNA library was hybridized to the Human Exome 2.1M Array (Nimblegene 05-547-792-001) for exome enrichment and then subject to Illumina GAII or HiSseq sequencing. Approximately 120 million 90 bp reads were generated for each sample, corresponding to an average sequencing depth of ~ × 250 for the exome. The reads were mapped to hg19 (UCSC) by bowtie2 with default settings, and duplicated reads were removed by Picard. Single-nucleotide variants (SNVs) and indels were called on the GATK platform with default settings, and only those that passed all GATK filters were used. The resulting data were highly reliable, as evidenced by the fact that the vast majority of variants called at a given stage were also found at later stages. All SNVs and indels genotyped as 0/1 or 1/1 in MCF10A or MCF10A- HRAS were considered germ-line SNPs or indels and were excluded from further analyses. These data are presented in Supplementary Data 2 . The raw data have been deposited into GEO with the accession numbers of GSE63630 and PRJNA268433 . Poly(A) + RNA sequencing Total RNA was extracted from ~3 × 10 6 cells using the RNeasy Kit (Qiagen 74134,79654), followed by DNase I (Promega RQ1 RNase Free DNase) treatment to eliminate DNA contamination. Samples with an RNA integrity number (RIN) >9.5 (Agilent 2100 Bioanalyzer) were used. Poly(A) + mRNA was isolated with Dynabeads Oligo(dT) 25 (Life Technology 61005). Libraries were constructed following the TruSeq RNA Guide (Illumina) and subject to Illumina GAII or HiSseq sequencing. Approximately 20 million 75 bp reads were generated for each sample. The RNA-seq reads were mapped to hg19 (UCSC) by bowtie2 with default settings. Reads with mapping quality higher than 20 that mapped to exon regions (Ensemble 69) were considered unique hits. For genes with alternative splicing, only exons from the longest transcript were considered. The RPKM of a gene was calculated similarly to a previous study [42] . The effective length of a gene was defined as the total number of the 75-mers in all its exons that hits nowhere else in the genome. We excluded genes with effective length <100 bp from subsequent analyses. These data are presented in Supplementary Data 3 . Separation of intratumoural subclones We started with the 8081 substitution mutations that were sequenced with > × 30 coverage in all samples. We excluded 7,608 sites that were annotated as the same genotype by GATK in all XT samples to simplify the procedure of subclone separation. The remaining 473 sites were hierarchically clustered according to their mutant allele frequencies, which often varied at different tumour stages. We observed 72 sites showing mutations specifically in XT8_M1, while among the rest of the mutations, we identified four major groups together representing diverse subclones. There were 15 sites that could not be reliably grouped. The relationships of the mutation groups were resolved by reasoning and further experimental validation. To define a mutation present at a specific stage, we required that the mutant allele frequency be >1%. We defined copy-number neutral regions with no loss of heterozygosity as frequency informative regions (FIRs). The cell frequency of a subclone is two times the average of allele frequencies of the mutations found in the subclone and located at FIRs. We used serial dilution to obtain single cells that were seeded onto 96-well plates. Microscopic observation confirmed those wells that contained only one cell. At a very low frequency (<1%), we obtained small colonies each consisting of at least a few dozen cells in a well. Genomic DNA was extracted from such colonies and then used for assessment of intratumoural subclone separation. These data are presented in Supplementary Data 2 . Analysis of mutations found in XT8 and the metastases For each of the four mutations there was a neighbouring germline single-nucleotide polymorphism (SNP) that identifies the two alleles of the locus. High-fidelity polymerase chain reactions (PCR) followed by TA cloning and Sanger sequencing were performed in XT8_M1 and XT8_M2, respectively, to trace the allele information of the mutations. These data are presented in Supplementary Fig. 3 . Detection of positive selection All mutation data from clinical cancer samples were retrieved from TCGA [43] and COSMIC [44] . The mutation spectrum of breast cancer was determined by analysing substitution mutations in breast cancer exomes sequenced by TCGA, with only fourfold degenerate sites of protein-coding genes considered. Using the breast cancer mutation spectrum, we then computed the numbers of non-synonymous (missense and nonsense) and synonymous sites of the merged coding sequences of the 14 multicellularity-related genes to estimate their d N and d S in the breast cancer clinical samples. We examined the locations and neighbouring bases for all of the non-synonymous and nonsense mutations of the 14 genes observed in the xenograft tumours and clinical samples, and confirmed that the high d N / d S ratios cannot be explained by a few extremely biased mutation hotspots or certain biased mutation motifs. These data are presented in Supplementary Data 4 . Identification of putative driver expression changes We defined a gene with a marked expression change using two criteria: (1) there was more than a twofold difference between the maximum and minimal expression levels of the 12 samples; and (2) the difference is statistically significant at q <0.001 (Bonferroni correction). A total of 12,911 genes showed marked expression changes, with ~40% being predominantly downregulated (correlation coefficient R <0) during the tumour evolution. To define one-way expression divergence (or putative DEC), two rounds of analyses were perfomed, each with 11 cell samples (10 earlier samples and one of the two metastases) sorted according to their temporal order. For a gene with elevated (or reduced) one-way expression divergence three criteria had to be met: (1) its maximum expression among the 11 samples appeared later (or earlier) than its minimal expression; (2) for all pairwise comparisons, the earlier sample could not be higher (or lower) than the latter sample by >10% of the difference between the maximum and minimal expression levels; and (3) the above two criteria are met in both rounds of analyses where a different metastasis sample is examined. Among the 12,911 genes with marked expression changes, <6% (758) met these criteria. Fifty-five genes were completely silenced after HRAS transfection and thus were not considered because only the stochastic evolutionary process was of interest here; the remaining 703 genes were subject to further analyses. Correlation analysis revealed that ~75% of these genes were downregulated (indicated by the negative correlation coefficient between the ranking of evolution stages and the expression levels; R <0) during tumour evolution. These data are presented in Supplementary Data 3 . Dating the origin of human genes We included 13 major clades from single-celled organisms to non-human primates, considering previous reports [7] , [45] , [46] , [47] , [48] , [49] regarding the phylogeny, to trace the origin of 23,695 human protein-coding genes. The orthologous relationships between the human genes and genes of organisms in the 13 major clades were determined using OrthoMCL with default settings. For a given human gene, we first determined the most distant clade containing the gene’s orthologues and then assigned its birth to the latest common branch of human and that clade. To avoid potential age inflation due to horizontal gene transfer or unreliable orthology assignment, we required that the gene (or its orthologues) can be found in at least one additional clade, except for genes born at B12. Cases not satisfying this criterion were excluded, leaving 21,352 human genes, including 488 cancer drivers, with a birth time assigned. The birth rate of cancer drivers on a given branch was defined as the number of cancer drivers born on the branch divided by the total number of human genes born on the branch. As the completeness of the selected genomes in the 13 clades is critical, this parameter was evaluated using a previously described method [50] . In brief, a set of genes basic to all eukaryotes was used to query the selected genomes, with observation of 100% presence desired. We selected 36 species with sequenced genomes to represent the 13 clades, with a minimal completeness of ~96% at the clade Placozoa. Inclusion of more genomes did not improve the performance. The major point of this analysis lies in the three clades (Placozoa, Porifera and Ctenophora) representing early multicellular animals. To model the potential bias due to sparse sampling of the three clades, we performed 100 rounds of simulations by randomly removing 10% of genes of the genomes in each of the three clades and found that the overrepresentation of cancer genes at the Branch #3 remained qualitatively unchanged ( Supplementary Fig. 9 ). To control for protein evolutionary rate in the phylostratigraphy analysis, we sorted the 21,352 genes according to their d N between human and chimpanzee (The results were essentially the same when d N values between human and rhesus monkey were used. ), and then divided them into 100 equal-size bins (the fastest evolving bin has 213+52=265 genes). We randomly picked n genes from a bin, where n is the number of cancer drivers in the bin, to form a pseudo-cancer driver set with the 488 genes; the birth rate of the pseudo-cancer drivers on each of the 13 branches was then calculated. Such simulation was repeated 13,000 times to achieve a test at the significance level of P =0.01 after Bonferroni correction. The species and gene information are presented in Supplementary Data 6 . Novel tumour suppressors revealed by the d T / d S ratio test We downloaded TCGA level 3 data of substitution mutations from TCGA data portal. In total, 776 BRCA, 269 COAD, 291 GBM, 306 HNSC, 422 KIRC, 520 LUAD, 178 LUSC, 463 OV, 116 READ, 266 SKCM, 245 STAD, 406 THCA and 248 UCEC tumours were considered. For each cancer type we analysed the single-base substitution mutations at fourfold degenerate sites of protein-coding genes to derive the mutation spectrum of that cancer. In addition to the six regular types of substitution mutations, mutations of ApT->ApA, CpG->TpG and TpC->TpX (X: A, T and G), and TpCpG->TpTpG (the combination of TpC and CpG), were separately considered [22] . In other words, we computed the mutation rate U for each of the 12 mutation types in each cancer to estimate the expected truncating versus synonymous (T/S) site ratio of a gene. For a hypothetical gene with two codons, for example, TACTGC, there are 18 mutation possibilities: aACTGC, cACTGC, aACTGC, TtCTGC, TcCTGC, TgCTGC, TAaTGC, TAtTGC, TAgTGC, TACaGC, TACcGC, TACgGC, TACTaC, TACTtC, TACTcC, TACTGa, TACTGt and TACTGg (only one-step mutations are considered because of the low mutation rate). For each mutation possibility the expected rate is the U of the corresponding mutation type. We then compute the summed expected rate ( U ) for truncating mutation possibilities (here, TAaTGC, TAgTGC and TACTGa) and synonymous mutation possibilities (here, TAtTGC and TACTGt), and the expected T/S site ratio is the former divided by the latter. The d T / d S ratio is the observed T/S mutation ratio divided by the expected T/S site ratio. Multiple testing was controlled using the method of Storey [51] . These data are presented in Supplementary Table 3 . Software or URLs. Bowtie2 (ref. 52 ) for short reads mapping; Picard ( http://picard.sourceforge.net ) for removing duplicated short reads; GATK [53] for SNVs and indels calling; Cluster 3.0 (ref. 54 ) for clustering analysis; R-package affy [55] for microarray data processing; BinGO [56] and GSEA for Gene Ontology analysis; ENSEMBL http://asia.ensembl.org ; UCSC hg19 http://genome.ucsc.edu ; ENCODE http://genome.ucsc.edu/ENCODE/ ; Bodymap 2.0 http://www.ncbi.nlm.nih.gov/geo/query/acc.cgi?acc=GSE30611 ; GO http://www.geneontology.org/;TumorScape http://www.broadinstitute.org/tumorscape ; OrthoMCL http://orthomcl.org/orthomcl/ . How to cite this article: Chen, H. et al . The reverse evolution from multicellularity to unicellularity during carcinogenesis. Nat. Commun. 6:6367 doi: 10.1038/ncomms7367 (2015).